Genome-wide association study identifies new susceptibility loci for epithelial ovarian cancer in Han Chinese women Ovarian cancer is the leading cause of death from gynaecological malignancies worldwide. Here we perform a three-stage genome-wide association study (GWAS) in Han Chinese women to identify risk genetic variants for epithelial ovarian cancer (EOC). We scan 900,015 single-nucleotide polymorphisms (SNPs) in 1,057 EOC cases and 1,191 controls in stage I, and replicate 41 SNPs ( P meta <10 −4 ) in 960 EOC cases and 1,799 controls (stage II), and an additional 492 EOC cases and 1,004 controls (stage III). Finally, we identify two EOC susceptibility loci at 9q22.33 (rs1413299 in COL15A1 , P meta =1.88 × 10 −8 ) and 10p11.21 (rs1192691 near ANKRD30A , P meta =2.62 × 10 −8 ), and two consistently replicated loci at 12q14.2 (rs11175194 in SRGAP1 , P meta =1.14 × 10 −7 ) and 9q34.2 (rs633862 near ABO and SURF6 , P meta =8.57 × 10 −7 ) ( P <0.05 in all three stages). These results may advance our understanding of genetic susceptibility to EOC. Ovarian cancer is one of the most common cancers among women and the leading cause of deaths from gynaecological malignancies in the world [1] . In addition to familial BRCA1 and BRCA2 mutations, there are other kinds of genetic risk factors, including common genetic variants of lower penetrance [2] , [3] . Molecular epidemiological studies have been conducted with the candidate gene approach to identify low penetrance susceptibility genes for ovarian cancer, many of which have showed inconsistent results [4] , [5] , [6] , [7] , [8] , [9] , [10] , [11] . Recent genome-wide association studies (GWASs) have reported 11 new single-nucleotide polymorphisms (SNPs) that are associated with ovarian cancer risk in European populations [12] , [13] , [14] , [15] , [16] , [17] . However, the results from the published GWASs have also demonstrated race- and ethnicity-specific cancer susceptibility [18] . Therefore, additional GWASs are needed to identify new ovarian cancer susceptibility genes, especially in non-European populations. Here we report a three-stage GWAS that identifies new common genetic variants associated with ovarian cancer risk in Han Chinese women. We identify two SNPs that are significantly associated with ovarian cancer risk (rs1413299 in COL15A1 , P meta =1.88 × 10 −8 and rs1192691 near ANKRD30A , P meta =2.62 × 10 −8 ) in Chinese women and two other consistently replicated loci (rs11175194 in SRGAP1 , P meta =1.14 × 10 −7 and rs633862 near ABO and SURF6 , P meta =8.57 × 10 −7 ). In addition, we also confirm rs9303542 at 17q21 from those 11 SNPs in previously reported GWASs of the Europeans. 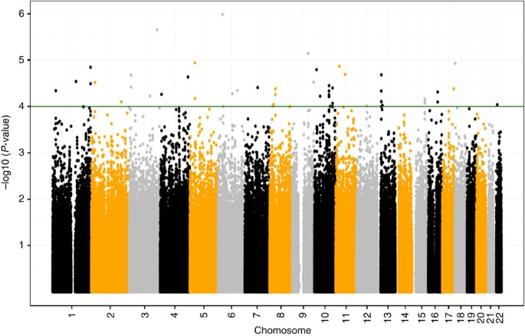Figure 1: Genome-wide association results for EOC in Han Chinese women. Manhattan plot showing the genome-wide association results for ovarian cancer. The association between 710,714 genotyped SNPs and ovarian cancer risk (1,044 ovarian cancer cases and 1,172 controls) was analysed. The green horizontal line representsP=1.0 × 10−4. Association analyses We conduct a three-stage GWAS in Han Chinese women ( Table 1 and Supplementary Table 1 ). In the initial discovery stage, we perform a GWA scan in 1,057 epithelial ovarian cancer (EOC) cases and 1,191 age-matched healthy controls using the Illumina HumanOmniZhongHua-8 BeadChip, which contains 900,015 SNPs. After the standard quality control (QC) filtering, 710,714 SNPs and 2,216 individuals (1,044 cases and 1,172 controls) are included in the follow-up analyses ( Supplementary Fig. 1 ). Principal component analysis (PCA) shows little evidence of population stratification in each (northern and southeastern) of the GWA scan populations (see Methods and Supplementary Fig. 2 ). We use logistic regression with adjustment for age and the first three eigenvectors to test the additive effect of a minor allele of each SNP. Meta-analysis was used to combine the results of the two populations in the GWA scan. Table 1 Three-stage study design of ovarian cancer GWAS in Chinese women. Full size table For the replication in stage II, we genotype 41 SNPs in an independent sample set of 960 EOC cases and 1,799 controls ( Fig. 1 and Supplementary Data 1 ). The selection criteria of 41 SNPs were described in Methods. 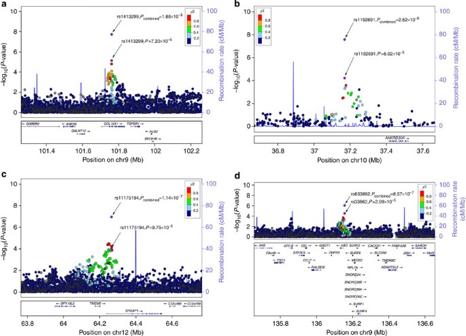Figure 2: Regional plots of the four ovarian cancer susceptibility loci. Regional plots of four newly discovered loci associated with the risk of ovarian cancer in Chinese women in the GWAS discovery stage. The results (−log10P,P-value of the meta-analysis for all populations) are shown for SNPs in the region 500 kb up- or downstream of the marker SNP. The marker SNPs are shown as purple circle in stage I and as purple diamonds in combined stages; the LD values (r2) between that SNPs and the most strongly associated SNP (diamond) are indicated by the heat scale. The genes within the region of interest are annotated and the directions of transcripts are shown in arrows. As a result, four SNPs associated with a significant cancer risk in stage II (rs1413299 ( P meta =4.00 × 10 −3 ) at 9q22.33, rs1192691 ( P meta =3.00 × 10 −3 ) at 10p11.21, rs11175194 ( P meta =3.58 × 10 −3 ) at 12q14.2 and rs633862 ( P meta =2.38 × 10 −2 ) at 9q34.2) ( P meta <0.05) were further subjected to replication in stage III and consistently validated ( Table 2 ). In the combined analysis of the five substudies (that is, Ia, Ib, IIa, IIb and III) in all the three stages, two SNPs (rs1192691, odds ratio (OR)=0.81, 95% confidence interval (CI)=0.75–0.87, P meta =2.62 × 10 −8 and rs1413299, OR=1.24, 95% CI=1.15–1.33, P meta =1.88 × 10 −8 ) reached the genome-wide significance ( P <5 × 10 −8 ) without significant heterogeneity among all the stages. In addition, the other two consistently validated ( P <0.05 in all the three stages) SNPs also showed strong associations but short of the genome-wide significance (rs11175194, OR=0.82, 95% CI=0.76–0.88, P meta =1.14 × 10 −7 and rs633862, OR=0.83, 95% CI=0.77–0.89, P meta =8.57 × 10 −7 ) ( Table 2 and Supplementary Fig. 3 ). These four SNPs have not reported in the previous GWASs of the Europeans, possibly due to racial diversity and differences in study power. For example, the minor allele frequency (MAF) of these four SNPs was quite different between European and Asian populations in the HapMap project ( http://hapmap.ncbi.nlm.nih.gov/ ). In the previous GWASs, only a limited number of top-hit SNPs were validated in a large sample size. Therefore, additional GWASs need to be performed in other non-European populations. Figure 1: Genome-wide association results for EOC in Han Chinese women. Manhattan plot showing the genome-wide association results for ovarian cancer. The association between 710,714 genotyped SNPs and ovarian cancer risk (1,044 ovarian cancer cases and 1,172 controls) was analysed. The green horizontal line represents P =1.0 × 10 −4 . Full size image Table 2 Summary of GWAS scan and replication studies for the four SNPs. Full size table Stratification analyses by histological subtype We then evaluated the associations between these four SNPs and EOC risk after stratifying cases by histological subtype. We found no evidence of significant heterogeneity among the subtypes ( Table 3 ). Using the imputation analyses based on data from the 1,000 Genomes Project (Phase I integrated variant set release, v3, http://www.1000genomes.org/ ), we tested for the risk associations of the SNPs (imputed info >0.5, MAF≥0.05) surrounding the lead SNPs in a 500-kb window, and we observed a series of significant signals around rs1413299 at 9q22.33 and rs11175194 at 12q14.2 ( Supplementary Table 2 and Fig. 2 ). Table 3 Ovarian cancer risk associated with the four identified SNPs in stratified analysis by histological subtype. Full size table Figure 2: Regional plots of the four ovarian cancer susceptibility loci. Regional plots of four newly discovered loci associated with the risk of ovarian cancer in Chinese women in the GWAS discovery stage. The results (−log10 P , P -value of the meta-analysis for all populations) are shown for SNPs in the region 500 kb up- or downstream of the marker SNP. The marker SNPs are shown as purple circle in stage I and as purple diamonds in combined stages; the LD values ( r 2 ) between that SNPs and the most strongly associated SNP (diamond) are indicated by the heat scale. The genes within the region of interest are annotated and the directions of transcripts are shown in arrows. Full size image We also evaluated the associations for SNPs in stage I with serous ovarian cancer risk, the dominant histologic subtype. We found that 104 SNPs were significantly associated with cancer risk among 594 patients with serous ovarian cancers and 1,172 controls ( P meta <1.00 × 10 −4 ). Of these 104 SNPs, 21 SNPs were also significantly associated with overall risk of ovarian cancer, and rs6784988 ( P serous =3.57 × 10 −7 ; P total =2.23 × 10 −6 ) at 3q26.33 and rs7420064 ( P serous =3.87 × 10 −7 ; P total =4.04 × 10 −6 ) at 2q13 were the top hits ( Supplementary Data 2 ). Further validation studies are warranted to confirm these SNPs in large populations. Association analyses of previously reported SNPs Previous GWASs of ovarian cancer have reported a number of SNPs that were associated with ovarian cancer risk among populations with a European ancestry [12] , [13] , [14] , [15] , [16] , [17] . The present study in Han Chinese populations also tested the risk associations with the 11 previously reported SNPs from those GWAS analyses, but only 8 SNPs were included in our GWA scan or imputation analyses, of which four SNPs (rs2665390 at 3q25, rs9303542 at 17q21, rs8170 at 19p13.11 and rs757210 at 17q12) were found to be significantly associated with EOC risk in our stage I study. We successfully re-designed the primers for 10 of the 11 SNPs and genotyped them in our stage II and III studies, and we identified 1 SNP (rs9303542 at 17q21) that was significantly associated with EOC risk ( Supplementary Table 3 ) in both stage I and replication data sets. This rs9303542 SNP is intronic to SKAP1 , which has strong homology to SRC oncogene at the carboxy-terminal end of their proteins. Although not significantly replicated, all of the tested SNPs were in the same direction of ORs published in previous GWASs. These discrepant results are probably due to the relatively lower statistical power of the present study and racial diversity. Molecular analyses The SNP may exert a long-range effect on the expression of genes upstream and downstream of the loci. A search of genes that were present within 1 Mb of the SNP revealed some potentially interesting genes ( Fig. 2 and Supplementary Table 4 ). To gain further insight for the possible involvement of these genes in ovarian cancer pathophysiology, we examined whether expression levels of these genes are clinically relevant by using the comprehensive data from The Cancer Genome Atlas. Interestingly, these gene expression data suggested that COL15A1 ( P =3.03 × 10 −3 ) gene expression levels were significantly different between tumours and normal tissues, and that the expression levels of TGFBR1 (transforming growth factor-β receptor type I) were also significantly associated with patient survival ( P =7.00 × 10 −4 ). ANKRD30A expression data from The Cancer Genome Atlas suggested that there was no significant difference in the expression levels between ovarian cancer and normal tissues. In this three-stage GWAS of EOC, we identified two SNPs that were significantly associated ( P <5 × 10 −8 ) with ovarian cancer risk in Chinese women and two other consistently replicated ( P <5 × 10 −7 ) loci. The top-signal SNP, rs1413299, is in intron 6 of COL15A1 that encodes the α-chain of type XV collagen at 9q22.33, a member of the FACIT (fibril-associated collagens with interrupted helices) collagen family. Loss of the COL15A1 protein from the basement membranes/basement membrane zone was reported to promote tumour cell infiltration in human ductal breast carcinoma cells and colon carcinomas [19] , [20] . In addition, COL15A was found to suppress tumorigenesis in a dose-dependent manner in human cervical carcinoma cell line [21] . Interestingly, rs1413299 is located in the DNase-seq, Chip-seq and Histone modification peak regions in dozens of cell lines, including lymphocyte-derived cell lines (GM12878) and breast cell lines (MCF-7; data from the Encode project, http://genome.ucsc.edu/ENCODE/ ) [22] , indicating its potential biofeatures of an enhancer. By querying results from CTCF ChIA-PET in the Encode Project [23] , [24] , we further found interaction signals in the region and nearby genes ( TGFBR1 and GALNT2 ) in MCF-7, suggesting possible putative distant chromatin interactions bounded by CTCF. TGFBR1 is located 105 kb downstream of rs1413299, which is a central propagator of the TGF-β signalling pathway that is an important regulator of several important biological processes, including cell proliferation, differentiation, migration, apoptosis and matrix accumulation [25] . Participating in the activity of the TGF-β signalling pathway [26] , [27] , TGFBR1 binds to TGF-β and forms a heterodimeric complex with TGFBR2, leading to phosphorylation and activation of SMAD2 and SMAD3. Furthermore, TGFBR1 expression was found to be markedly reduced in recurrent ovarian tumours [28] . In addition, the deletion of TGFBR1 * 6A/9A, which was known to be associated with risk of multiple cancers, was also reported to be associated with ovarian cancer risk [29] , [30] . Therefore, additional studies are warranted to explore a possible role for TGFBR1 in the aetiology of EOC and a potential mechanistic link between rs1413299 and the functions of TGFBR1 . Thus, we hypothesized that rs1413299 variants may have a different expression pattern of downstream genes through a long-range chromatin interaction and eventually influence the risk of ovarian cancer. The second identified SNP, rs1192691, is located 245 kb upstream of exon 1 of ANKRD30A that encodes the ankyrin repeat domain 30A, and this gene is also known as NY-BR-1 . NY-BR-1 is a breast cancer differentiation antigen and a potential target for cancer immunotherapy [31] . No associations with EOC risk and functional implications of NY-BR-1 in EOC have been reported in previous ovarian cancer studies; however, the oestrogen-response element-like sequences nearby the NY-BR-1 promoter region suggests that the NY-BR-1 expression may be regulated through oestrogen receptors [32] . Additional studies are warranted to further understand the implication of this gene in ovarian cancer. The third SNP, rs11175194, is located in the first intron of SRGAP1 that encodes the SLIT-ROBO Rho GTPase-activating protein 1. The Rho family small GTPases serve as molecular switches involved in several cellular progresses [33] . It is reported that overexpression of Rho GTPases in cancers was correlated with poor prognosis [34] and that SNPs in the SRGAP1 gene were associated with papillary thyroid carcinoma [35] . As a subfamily of Rho GTPase-activating proteins, SRGAP1 is involved in regulation of the RhoA activity through interacting with CDC42 that has been proven to exert an important role in cancer development [36] . Interestingly, CDC42-positive macrophages may prevent malignant transformation of ovarian endometriosis [37] . The fourth SNP, rs633862, is located 5 kb upstream of ABO (ABO blood group). ABO determines the ABO blood group of an individual by modifying the oligosaccharides on cell surface glycoproteins. This SNP has a moderate linkage disequilibrium (LD) with rs8176719 ( r 2 =0.57, CHB (Han Chinese in Beijing) population in the 1,000 genome project), an SNP also named the O allele frame-shift mutation affecting amino acid 176. Furthermore, the minor allele of rs633862, suggested the O subgroup, has been found to exert a protective role in ovarian cancer risk in the present study, which is consistent with the findings of previously published studies: A and B subgroups were associated with modestly increased risk of ovarian cancer [38] , [39] , [40] . In summary, in this GWAS of Han Chinese women on EOC susceptibility, we definitively (at P <5 × 10 −8 ) identified two new susceptibility loci at 9q22.33 and 10p11.21, and two other consistently replicated (at P <5 × 10 −7 ) loci at 12q14.2 and 9q34.2. In addition, we also confirmed 1 locus at chromosome 17q21 from those 11 SNPs in previously reported GWASs of the Europeans. Further studies with larger sample sizes are warranted to replicate our findings. Fine mapping around these new loci and related functional studies should be carried out to elucidate the underlying mechanism for the observed associations. Study populations We performed a three-stage GWAS in Han Chinese women for EOC susceptibility. A summary of all cases and controls in the study is provided in Supplementary Table 1 . The GWA scan phase included 1,044 EOC patients and 1,172 controls (429 cases and 425 controls from Northern Chinese, and 615 cases and 747 controls from Southeastern Chinese), followed by two stages of validation (stage II: 408 cases and 900 controls of Southern Chinese; 552 cases and 899 controls of Southeastern Chinese, and stage III: 492 cases and 1,004 controls of Northern Chinese). There were six studies that were included in this three-stage study. Northern Chinese population was from TOCS (Tianjin Ovarian Cancer study), CAMSCH (Chinese Academy of Medical Sciences Cancer Hospital) and BUCT (Beijing University of Chemical Technology). Southeastern Chinese population was from NOCS (Nanjing Ovarian Cancer study) and SOCS (Shanghai Ovarian Cancer study). Southern Chinese population was from GOCS (Guangzhou Ovarian Cancer study). All EOC cases were recruited in local hospitals and had the pathologically proven disease. Cancer-free controls were recruited in local hospitals for individuals receiving routine physical examinations or in the communities for those participating in the screening of non-communicable diseases. The cases and controls were frequency-matched for age in both the GWA scan stage and validations. At recruitment, informed consent was obtained from each subject, and this study was approved by the institutional review boards of each participating institution. The TOCS enrolled patients with newly diagnosed and histologically confirmed EOC from Tianjin Medical University Cancer Hospital in Tianjin, China. Patients with a previous medical history of cancer, or previous radiotherapy or chemotherapy were excluded. Controls were recruited from cancer-free subjects who underwent regular health check-up during the same time when cases were recruited, and lived in the same neighbourhoods or nearby communities. The controls were frequency-matched to cases on age. All subjects were ethnic Chinese. The study was approved by the Committee on Human Research of Tianjin Medical University Cancer Hospital. The CAMSCH study recruited cases from Beijing city and surrounding provinces of Beijing. The eligible patients with newly diagnosed, histopathologically confirmed and previously untreated (by radiotherapy or chemotherapy) ovarian cancer were accrued between January 2009 and June 2012 at the Cancer Hospital, Chinese Academy of Medical Sciences. All participants were of unrelated Han Chinese ethnicity. Each patient was interviewed for detailed information on demographic characteristics and lifestyles. Controls were recruited from the TOCS and were frequency-matched to cases on age. The study was approved by the Committee on Human Research of Cancer Hospital, Chinese Academy of Medical Sciences. The BUCT enrolled cases and controls from the Shandong area of China. Cases were incident patients diagnosed with ovarian cancer at the Shandong Cancer Hospital. All of the cases had histologically confirmed ovarian cancer. Controls were healthy, cancer-free subjects selected from health examination clinics of the same hospital. All subjects were ethnic Chinese. The study was approved by the Committee on Human Research of Beijing University of Chemical Technology. The NOCS EOC cases were recruited from Jiangsu Provincial Hospital of Traditional Chinese Medicine and Nantong Tumor Hospital, southeastern China. The criteria for the recruitment of EOC cases included: (1) Han Chinese; (2) without previous malignant tumours in any other organs; and (3) histopathologically confirmed diagnosis. Cancer-free controls were randomly selected from the health examination clinics of the same hospitals during the same time period of case recruitment and were frequency-matched to cases by age. Each individual was interviewed face-to-face by trained interviewers to get information on demographic characteristics and lifestyles. The study was approved by the Committee on Human Research of Nanjing Medical University. The SOCS recruited cases from two hospitals, of which 1,167 ovarian cancer cases were consecutively recruited between March 2009 and August 2012 from Fudan University Shanghai Cancer Center (FUSCC), and the other 159 ovarian cancer cases were consecutively recruited between March 2012 and August 2012 at the Jiangsu Cancer Hospital (JCH). All tumours were histopathologically confirmed independently as primary epithelial ovarian carcinoma by two gynaecologic pathologists as routine diagnosis at FUSCC or at JCH. During an in-person interview, all potential subjects provided information about their demographics and known risk factors. The study was approved by the Committee on Human Research of Fudan University Shanghai Cancer Center. The GOCS enrolled case and controls from Guangdong area of China. Cases were the EOC patients who underwent tumour resection between 2002 and 2012 in Sun Yat-sen University Cancer Center. The diagnosis was confirmed histologically in all cases. Controls were recruited from subjects who underwent regular health check-up during the same time period of cases in several cities including Guangzhou, Zhongshan and Sihui, and matched by age. The study was approved by the Committee on Human Research of Sun Yat-sen University Cancer Center. Genotyping and QC in the GWAS We genotyped a total of 900,015 SNPs in the GWA scan with 1,057 cases and 1,191 controls by using Illumina HumanOmniZhongHua-8 BeadChip. Before the association analysis, a systematic QC procedure was applied to the raw genotyping data to filter both unqualified SNPs and samples (see flow diagram in Supplementary Fig. 1 ). We excluded SNPs from further analysis if they (1) did not map to autosomal chromosomes; (2) had a low call rate in GWAS samples (<95%); (3) had MAF<0.05; and (4) were deviated from Hardy–Weinberg equilibrium ( P <1.0 × 10 −5 ). We also removed individuals from further analysis if they (1) had an overall successful genotyping call rate<95%; (2) had sex discrepancies between the records and the genetically inferred data; and (3) were the unexpected duplicates or probable relatives (all PI_HAT>0.25). We detected population outliers by using a method based on PCA. A set of 106,963 common autosomal SNPs (MAF>0.25) with low LD ( r 2 <0.20) were used to identify population outliers in the samples that had passed QC, using the founders of the HapMap trios of Yoruba in Ibadan ( N =90), Utah residents of Northern and Western European ancestry ( N =90), CHB (Han Chinese in Beijing) ( N =45) and JPT (Japanese in Tokyo) ( N =44) as the internal controls ( Supplementary Fig. 2 ). The PCA showed that the cases and controls were genetically matched in both the Northern and Southeastern Chinese populations ( Supplementary Fig. 2 ), and the genomic control inflation factor ( λ ) were 1.028 and 1.015, respectively, after adjustment for the first three principal components. After the QC process, a total of 1,044 cases and 1,172 controls with 710,714 SNPs were included in further analyses. SNP selection and genotyping in the replication studies We selected SNPs from the GWA scan phase for the stage II analysis based on the following criteria: (i) P meta <1.0 × 10 −4 ; (ii) the same association direction between Northern and Southeastern studies; and (iii) only the SNP with the lowest P -value was selected when multiple SNPs were observed but in strong LD ( r 2 ≥0.8). Eight SNPs met the criteria for replication, but those that had a strong LD ( r 2 >0.8) with the selected SNPs were not included in replication ( Supplementary Table 5 ). The SNPs that were significantly associated with EOC risk in the stage II analysis ( P <0.05) were further genotyped in stage III samples using Taqman. Genotyping in stages II and III was performed using the iPLEX MassARRAY platform (Sequenom, Inc.) of the 41 SNPs. The primers and probes are available on request. Laboratory technicians who performed genotyping experiments were blinded to case or control status. Five per cent of the samples were randomly selected for repeated genotyping as blind duplicates, and the reproducibility was 100%. Statistical analysis Associations between SNP genotypes and disease status were assessed in an additive model in PLINK v1.07 ( http://pngu.mgh.harvard.edu/~purcell/plink/ ) using logistic regression modeling (1 degree of freedom) with adjustment for age and the first three principal components. For the meta-analysis, a fixed-effects model was used when the Cochran’s Q statistic showed no heterogeneity ( P for Q >0.05); otherwise, a random-effects model (DerSimonian–Laird) was applied. Specifically, for the selection of SNPs used in the stage II analysis, we used the fixed-effects model that allowed us to include more candidate SNPs. Population structure was evaluated by the PCA in the software package EIGENSTRAT 4.2, and Manhattan plot of –log 10 P was generated using package ggplot2 in R 2.15.1 ( http://www.r-project.org./ ). The chromosome regions were plotted using an online tool, LocusZoom 1.1 ( http://csg.sph.umich.edu/locuszoom/ ). We used the Shapeit v2 (Phasing step, http://www.shapeit.fr/ ) and IMPUTE2 (Imputation step) software ( http://mathgen.stats.ox.ac.uk/impute/impute_v2.html ) to impute untyped SNPs using the LD information from the 1000 Genomes Project (Phase I integrated variant set release, v3, across all 1,092 individuals, http://www.1000genomes.org/ ) and imputed SNPs were with info score >0.8. All other analyses were performed using R 2.15.1. How to cite this article: Chen, K. et al. Genome-wide association study identifies new susceptibility loci for epithelial ovarian cancer in Han Chinese women. Nat. Commun. 5:4682 doi: 10.1038/ncomms5682 (2014).